Hawks steer attacks using a guidance system tuned for close
pursuit of erratically manoeuvring targets Aerial predators adopt a variety of different hunting styles, with
divergent flight morphologies typically adapted either to high-speed interception or
manoeuvring through clutter, but how are their sensorimotor systems tuned in
relation to habitat structure and prey behavior? Falcons intercept prey at
high-speed using the same proportional navigation guidance law as homing missiles. This classical guidance law works well in the open, but performs sub-optimally
against highly-manoeuvrable targets, and may not produce a feasible path through the
cluttered environments frequented by hawks and other raptors. Here we identify the
guidance law of n = 5 Harris’ Hawks Parabuteo unicinctus chasing erratically manoeuvring
artificial targets. Harris’ Hawks use a mixed guidance law, coupling low-gain
proportional navigation with a low-gain proportional pursuit element. This guidance
law promotes tail-chasing and is not thrown off by erratic manoeuvres, making it
well suited to the hawks’ natural hunting style, involving close pursuit of agile
prey through clutter. The relationship between form and function is nowhere clearer than in
the morphology, physiology and behaviour of aerial predators—from the echolocation
systems of bats, to the streamlined silhouette of a stooping raptor. Birds of prey
adopt a range of hunting styles shaped by habitat structure, prey behaviour and
flight performance [1] : hawks have broad, lightly loaded wings that
enable them to turn quickly during short surprise attacks through clutter, whereas
falcons have narrower and more heavily loaded wings suited to fast long-range
attacks in open environments [2] . Flight performance is only a part of the
story, however, because attack success also hinges on the feedback system used to
guide flight after evasive prey [3] . The higher-level clades containing hawks and
falcons diverged >60 mya, but as their common ancestor with other landbirds is
also thought to have been an apex predator [4] , [5] , it is reasonable to suppose that their raptorial
guidance systems might share a common evolutionary origin. In level flight,
Peregrine Falcons Falco peregrinus have recently
been shown to use the same proportional navigation guidance law as
missiles [6] , which commands turning in proportion to the
angular rate of the line-of-sight from attacker to target [7] . At high enough gain, this
feedback system produces an attack trajectory called a parallel navigation (or
constant absolute target direction, CATD) course, in which the geographic direction
of the line-of-sight remains approximately constant, causing the attacker to
intercept its target by heading it off. This is in contrast to the simpler geometry
of a pure pursuit course, in which flight is always aimed directly at the target,
causing the attacker to follow its target in a tail-chase. Hawks may be expected to
use a different guidance law to Peregrine Falcons in level flight, because their
attacks have been found to involve a mixture of different guidance behaviours,
combining elements of parallel navigation with elements of pure
pursuit [8] , although this work did not attempt to identify
the underlying feedback laws implementing these behaviours. Here we identify the guidance law of Harris’ Hawks Parabuteo unicinctus chasing erratically manoeuvring
artificial targets. The hawks’ measured attack trajectories approximate a delayed
pure pursuit course, with flight directed at the location of the target after a
short lag. Such pursuit kinematics could be produced by one of several different
kinds of guidance law, including (i) proportional pursuit, in which turning is
commanded in proportion to the deviation angle between the attacker’s velocity
vector and its line-of-sight to target, and (ii) proportional navigation, in which
turning is commanded in proportion to the angular rate of the attacker’s
line-of-sight to target. In fact, we find that the dynamics are best modelled under
a mixed guidance law, in which turning is commanded by feeding back a linear
combination of the deviation angle and the line-of-sight rate with a small delay. Fitting the parameters of this mixed guidance law globally to all flights results in
a closer prediction of the observed flight behaviour than does fitting the
parameters of delayed proportional pursuit or delayed proportional navigation
independently to each flight. We conclude by discussing how the structure and tuning
of the hawks’ mixed guidance law relates to their typical hunting style involving
close pursuit of erratically manoeuvring targets, and consider how this compares
with the proportional navigation guidance law used during similarly level chases by
falcons specialised on hunting in open environments. 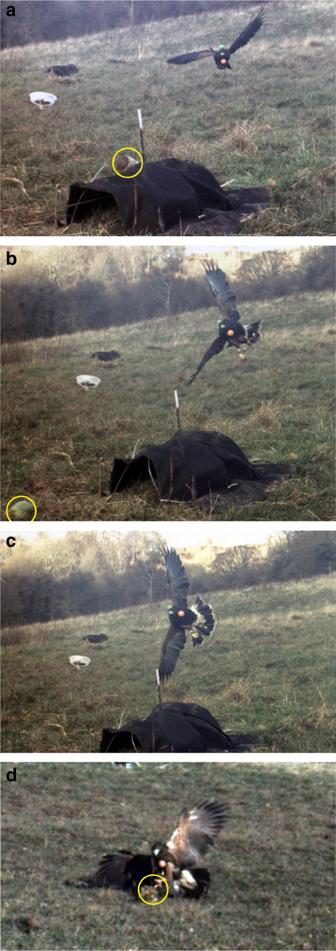Fig. 1 Sequence of video frames from a representative attack.
Five captive Harris’ Hawks chased a lure pulled at speed around
a randomised zigzagging course of pulleys and tunnels.aHawk initiating banked turn, with
its inside wing pitched down and its outside wing pitched up;bhawk at a high bank angle
0.25 s later, with its head held such that the eyes are
approximately level;chawk
fully banked another 0.05 s later, with its head still held with
the eyes approximately level;dhawk captures lure with one foot. Lure is circled yellow if
visible Experimental procedure We used four high-speed cameras recording at 250 Hz to reconstruct
the three-dimensional (3D) flight trajectories of n = 5 captive-bred Harris’ Hawks Parabuteo unicinctus (Supplementary Table 1 ) during 50 flights against an erratically
manoeuvring artificial target. The target comprised a food lure, which was towed
at speed around a series of pulleys to create a sequence of zigzagging turns
that we randomised on each trial to prevent the hawks from learning the course
(see Methods). The speed of the lure was adjusted continuously by the
experimenter (median lure speed: 7.0 m s −1 ;
interquartile range, IQR: 9.7 − 4.1 m s −1 ) to keep it
ahead of the hawk until the moment of capture. The resulting motions were
intended to mimic the erratic manoeuvres, or jinks, of a typical terrestrial
prey item (e.g. a hare or jackrabbit, Lepus spp.). There is very limited information available on typical prey performance,
and we did not attempt to model the behaviour of any particular prey item
specifically, but as a point of reference, the lure’s turning performance was
broadly comparable to that of a European Hare Lepus
europaeus , which has been recorded making a 60° evasive turn on a
7-m radius when fleeing a predator at
10 m s −1 [9] . Hawk attack kinematics approximate a delayed pure pursuit The hawks took off as soon as the lure began moving, flap-gliding to
reduce the range to their target. The birds banked to turn, whilst appearing to
keep their eyes level and their gaze directed at the target (Fig. 1a–c ; Supplementary Movies 1 and 2 ). The hawk rapidly extended one leg to capture the lure,
typically placing the other foot on the ground (Fig. 1d ). Because the recorded attack trajectories were always
close to planar, we projected them onto the two-dimensional (2D) ground plane
defined by the lure’s trajectory prior to further analysis. The hawks’ measured
track angle γ ( t ), defined as the bearing of their ground velocity vector in an
inertial frame of reference (Fig. 2a ),
was usually similar (Fig. 2b ) to their
line-of-sight angle λ ( t ), defined as the bearing of the position vector from hawk to
lure (Fig. 2a ). The linear association
between γ ( t ) and λ ( t ) was not always very strong, however
(Fig. 3a ), so to account for
expected sensorimotor delay, we also tried lagging the track angle by τ ≥ 0 (Fig. 3b ). The resulting correlation between γ ( t ) and λ ( t − τ ) for each flight
usually peaked at r > 0.8, given a small
delay with median value \(\tilde \tau = 0.16\) s (IQR: 0.22 − 0.12 s; here and elsewhere, tilde notation
denotes the median value of a parameter). It follows that the trajectories
approximated a delayed pure pursuit course, and not a parallel navigation
course, as is obvious also by inspection of the line-of-sight plots in
Fig. 2b . Although this simple
correlation analysis does not provide an explicit model of the dynamics, the
fitted delay is nevertheless comparable with the 0.13 s sensorimotor delay
fitted in a steering controller used to model pigeons negotiating
obstacles [10] . Fig. 1 Sequence of video frames from a representative attack. Five captive Harris’ Hawks chased a lure pulled at speed around
a randomised zigzagging course of pulleys and tunnels. a Hawk initiating banked turn, with
its inside wing pitched down and its outside wing pitched up; b hawk at a high bank angle
0.25 s later, with its head held such that the eyes are
approximately level; c hawk
fully banked another 0.05 s later, with its head still held with
the eyes approximately level; d hawk captures lure with one foot. Lure is circled yellow if
visible Full size image Fig. 2 Geometry of a pursuit. a Definition sketch showing: λ , the line-of-sight angle measured
between the line-of-sight (grey line) from hawk to target, and
some arbitrary inertial reference direction (dashed line); γ , the track angle
measured between the hawk’s velocity vector (blue arrow) and the
inertial reference direction (dashed line); δ , the deviation angle measured
between the line-of-sight from hawk to target (grey line), and
the hawk’s velocity vector (blue arrow). b 2D trajectory plots showing how the
instantaneous line-of-sight (grey line) between the hawk (blue)
and lure (magenta) varies through a flight for one randomly
selected flight per bird. Note that although the line-of-sight
is sometimes aligned with the direction of flight (as is
expected under the geometry of pure pursuit), the direction of
the line-of-sight itself is rarely held constant (as would have
been expected under the geometry of parallel navigation). Grid
spacing: 10 m Full size image Fig. 3 Correlation of track angle and line-of-sight angle. Each
figure panel plots a two-dimensional histogram of track angle γ against line-of-sight
angle λ for all sample points
over all flights: a no delay
between γ ( t ) and λ ( t ); b track angle γ lagged by τ = 0.16 s delay, representing the median value
of the delay at which the correlation between γ ( t + τ ) and λ ( t ) was maximised for each flight. The linear
association in b indicates that
the attack trajectories of the hawks approximated a delayed pure
pursuit course Full size image Attack dynamics are best modelled by a mixed guidance law The statement that the hawks’ attack trajectories approximated a
delayed pure pursuit course is agnostic with respect to the feedback system that
implements this. The simplest way to implement a pure pursuit course is to
command turning in proportion to the deviation angle δ = γ − λ between the velocity vector and the line-of-sight
to target (Fig. 2a ), such that \(\dot \gamma (t) = - K\delta (t - \tau )\) where K > 0 is a
guidance constant [7] . This proportional pursuit (PP) guidance law
drives δ to zero, so is a direct way of
implementing pure pursuit. An indirect approach is to use a proportional
navigation (PN) guidance law \(\dot \gamma (t) = N\dot \lambda (t - \tau )\) with its guidance constant set at N = 1, which commands turning at a rate \(\dot \gamma\) equal to the line-of-sight rate \(\dot \lambda\) , thereby holding δ = γ − λ unchanging [6] . This PN guidance law
differs fundamentally from PP, in that it has no tendency to drive δ to a specific value, so whereas both will produce
pure pursuit trajectories for δ (0) = 0, they
will produce different trajectories for other initial conditions. Yet another
possibility is to use a mixed guidance law \(\dot \gamma \left( t \right) = N\dot \lambda \left( {t - \tau } \right) - K\delta (t - \tau )\) combining PP and PN [7] , which has already been tested in several
other contexts in the missile literature [11] , [12] , [13] . To test between these alternatives, we
simulated all 50 flight trajectories under PP, PN and the mixed guidance law,
given knowledge only of the initial track angle and position of the hawk, and
the complete time history of both the lure’s motion and the hawk’s groundspeed
(Fig. 4 ). Fig. 4 Comparison of measured and simulated attack
trajectories. Panels display measured attack trajectories (dark
blue) and best-fitting simulations (light blue) for each Harris’
Hawk in pursuit of the lure (magenta), arranged by individual
bird (rows) and by guidance law (columns; PN: proportional
navigation; PP: proportional pursuit; PN + PP: mixed guidance
law). The time delay τ (s)
and guidance constant K (s −1 ) or N are independently fitted to each
flight for PP and PN, but are globally fitted to all flights for
the mixed guidance law. For each bird, we display the flight
with the least prediction error ε (m) under the mixed guidance law (excluding
flights <20 m), to best show the complementarity of its PN
and PP elements: whilst all flights are well-modelled by the
globally fitted mixed guidance law, some are not well-modelled
by PN or PP, despite these being independently fitted to each
flight; see Supplementary Figs. 1 – 9 for all other flights. Grid spacing: 10 m Full size image Because previous work on falcons had found variability in the
guidance constant between flights [6] , we began by fitting the time delay τ and guidance constant K or N for each
flight independently, minimising the prediction error ε , defined as the mean absolute distance between the measured
and simulated trajectories. To eliminate the attendant risk of overfitting, we
then tried fitting the parameters τ , K and N under the mixed guidance law to all flights together, holding
their values the same across all 50 flights. All three guidance laws were
capable of simulating the majority of the flight trajectories closely, when
fitting their guidance parameters independently to each flight. 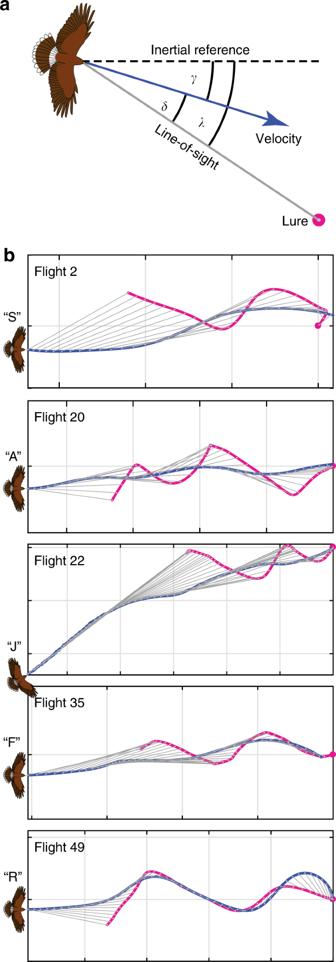Fig. 2 Geometry of a pursuit.aDefinition sketch showing:λ, the line-of-sight angle measured
between the line-of-sight (grey line) from hawk to target, and
some arbitrary inertial reference direction (dashed line);γ, the track angle
measured between the hawk’s velocity vector (blue arrow) and the
inertial reference direction (dashed line);δ, the deviation angle measured
between the line-of-sight from hawk to target (grey line), and
the hawk’s velocity vector (blue arrow).b2D trajectory plots showing how the
instantaneous line-of-sight (grey line) between the hawk (blue)
and lure (magenta) varies through a flight for one randomly
selected flight per bird. Note that although the line-of-sight
is sometimes aligned with the direction of flight (as is
expected under the geometry of pure pursuit), the direction of
the line-of-sight itself is rarely held constant (as would have
been expected under the geometry of parallel navigation). Grid
spacing: 10 m Beginning with
the two simplest guidance laws with only two fitted parameters per flight, the
median prediction error was \(\tilde \varepsilon = 0.46\) m for PP (IQR: 0.93 − 0.26 m; Bootstrapped 95% CI: 0.35,
0.70 m) and \(\tilde \varepsilon = 0.51\) m for PN (IQR: 0.96 − 0.19 m; Bootstrapped 95% CI: 0.32,
0.72 m), or just over 1% of the median distance flown (Supplementary
Table 2 ; Fig. 5a, d ). Fig. 5 Model parameters and fit under each guidance law. a – c proportional pursuit (PP), fitted
independently to each flight; d – f proportional navigation (PN), fitted independently to each
flight; g – i mixed (PP + PN) guidance law, fitted
independently to each flight; j – l mixed
(PP + PN) guidance law, fitted globally to all flights. a , d , g histograms
showing the prediction error ε of the best-fitting model for each flight,
where the solid and dashed red lines denote the median
prediction error \(\tilde \varepsilon\) and its bootstrapped 95% confidence interval; b , e , h histograms
showing the best-fitting guidance constant K (magenta) and/or N (blue) for each flight; c , f , i histograms
showing the best-fitting delay τ for each flight. j – l Surface
plots showing how median prediction error \(\tilde \varepsilon\) for all flights varies as a function of each
pair of the parameters N , K and τ of the mixed guidance law,
holding the third parameter constant at its best-fitting value. Surface colour denotes surface height; red dot denotes location
of global optimum Full size image The 50 independently fitted values of N followed a symmetric and well-behaved distribution
(Fig. 5e ), with a clear mode at N ≈ 1 as expected if the hawks had used
PN to implement pursuit ( \(\tilde N = 0.9\) ; IQR: 1.3 − 0.7). In contrast, the 50 independently fitted
values of K were highly skewed, with no clear
mode ( \(\tilde \tau = 0.00\) s −1 : IQR:
6.1 − 1.1 s −1 ; Fig. 5b ) and some extreme outliers (Supplementary
Table 2 ). The mean ranks of the
independently fitted values of N varied
significantly between individuals (Kruskal–Wallis test: χ 2 (4) = 12.96, p = 0.01), but a post hoc test found evidence of
only one significant pairwise difference between birds, so we do not attribute
much importance to this result. There was no evidence of any significant
variation in the independently fitted values of K between individuals (Kruskal–Wallis test: χ 2 (4) = 3.16 , p = 0.53). Interestingly, the majority of the PP
simulations entailed an effectively instantaneous response ( \(\tilde \tau = 0.00\) s; IQR: 0.09 − 0.00 s; Fig. 5c ), which in practice would imply the presence of a
predictive element to overcome the inevitable sensorimotor delay. In contrast,
the PN simulations typically involved a more delayed response, with a median
fitted delay of \(\tilde \tau = 0.10\) s (IQR: 0.19 − 0.00 s; Fig. 5f ), which is of similar magnitude to the sensorimotor delay
identified in previous studies of avian guidance
behaviours [10] . As most of the trajectories were well-modelled by either PP or PN,
we next asked whether these elements might be combined in a mixed guidance law. Because the mixed guidance law reduces to PP in the special case that N = 0, and reduces to PN in the special case that K = 0, it will inevitably model the data
at least as closely as either PP or PN if its guidance parameters are fitted to
each flight independently. When fitting this mixed guidance law independently to
each flight, the median prediction error was indeed significantly lower than for
either PP or PN, at \(\tilde \varepsilon = 0.18\) m (IQR: 0.36 − 0.09 m; Bootstrapped 95% CI: 0.13, 0.25 m;
Fig. 5g ), or <0.5% of the median
distance flown (Supplementary Table 2 ). Moreover, the populations of the independently fitted values
of N and K under the mixed guidance law followed a tighter and more symmetric distribution
( \(\tilde N = 0.7\) ; IQR: 0.8 − 0.4; \(\tilde K = 1.0\) s −1 ; IQR:
1.4 − 0.2 s −1 ; Fig. 5h ) than they did under either PP or PN (Fig. 3b, e ). Likewise, the median delay fitted under
the mixed guidance law was close to the delay of ~0.1 s fitted under PN, but
with a narrower spread ( \(\tilde \tau = 0.12\) s; IQR: 0.17 − 0.02 s; Fig. 5i ). The obvious difficulty with interpreting the results of
these independently fitted models is that they all risk overfitting to a greater
or lesser degree, with a total of 150 independently fitted parameters under the
mixed guidance model, and 100 independently fitted parameters for each of PP and
PN (see Supplementary Table 2 ). To eliminate the risk of overfitting completely, we therefore
searched for the unique combination of N , K and τ that minimized the median prediction error under the mixed
guidance law for all 50 flights simultaneously (Fig. 5j–l ). This mixed guidance law with just three globally
fitted parameters ( N = 0.7, K = 1.2 s −1 , τ = 0.09 s) had a median prediction error of \(\tilde \varepsilon =\) 0.34 m (bootstrapped 95% CI: 0.24, 0.53 m). Given that the
independently fitted PP and PN guidance laws, with 100 model degrees of freedom
each, had a higher median prediction error ( \(\tilde \varepsilon = 0.46\) m and \(\tilde \varepsilon = 0.51\) m, respectively), it is therefore reasonable to prefer the
globally fitted mixed guidance law with only 3 model degrees of freedom on
grounds of parsimony, despite the fact that the 95% CIs on the median prediction
error are overlapping. We conclude that the globally fitted mixed guidance law
provides the best balance between goodness of fit and model parsimony amongst
those we considered, closely capturing the observed turning behaviour on most of
the flights with only three fitted parameters (Figs. 4 , 5 ; Supplementary
Figs. 1 – 9 ). The sensorimotor feedback requirements of the PP and PN elements of
this mixed guidance law are quite different. Specifically, the deviation angle δ that is fed back under PP is the angle
between the velocity vector of the pursuer and its line-of-sight to target, and is
therefore defined egocentrically. This angle could be estimated in various ways, but
will be similar to the angle between the body axis and the sagittal plane if the
head is assumed to be kept level and to track the target closely. In contrast, the
line-of-sight rate \(\dot \lambda\) that is fed back under PN is defined in an inertial frame of
reference. Under the same set of assumptions on head tracking, the line-of-sight
rate could be estimated either by integrating the angular accelerations sensed by
the vestibular system, or by making direct use of the rotational optic flow cues
produced by the head’s self-motion relative to a fixed visual background. Feeding
back the line-of-sight rate as well as the deviation angle under a mixed guidance
law should improve the speed of response and reduce overshoot in a pursuit, because
the line-of-sight rate provides a prediction of how the deviation angle is changing. This is consistent with the observation that our best-fitting PP simulations
entailed effectively instantaneous sensory feedback (Fig. 3c ) requiring some form of prediction, in contrast to the
realistically delayed feedback that we found in the simulations fitted under PN
(Fig. 3f ) or the mixed guidance law
(Fig. 3i–k ). Why, though, should hawks tune their mixed guidance law to produce a
trajectory approaching a pure pursuit, rather than a parallel navigation course? Whereas the intercept trajectories associated with parallel navigation are
time-optimal against non-manoeuvring targets [7] , and may be nearly
time-optimal against manoeuvring ones [14] , the tail-chase trajectories associated with
pure pursuit are usually thought to be energetically costly and
inefficient [15] . It is an open question how these different
kinds of attack behaviours might perform in response to closed-loop evasive
manoeuvres. Pure pursuit has been observed in predatory cursorial
beetles [16] , [17] , but other aerial predators including
dragonflies [18] , [19] , flies [15] , [20] , bats [14] and
falcons [6] , [21] approximate a parallel navigation course. Previous research on another hawk species found a mix of
both [8] , which might be explained by the use of a mixed
guidance law combining elements of PP and PN. To understand the basis of this
interspecific variation, we must take a comparative approach to the dynamics. Conveniently, whilst the globally fitted mixed guidance law provides the more
parsimonious and marginally better-fitting model, a PN guidance law is capable of
describing our hawks’ measured attack trajectories nearly as closely if its
parameters are fitted independently for each flight, enabling phenomenological
comparison of their fitted N -values with those
of falcons (Fig. 6a ). Fig. 6 Comparative analysis of guidance behaviour. a Box-and-whisker plots comparing N -values for PN guidance
models fitted independently to 50 flights from Harris’ Hawks (this
paper) and 42 flights from Peregrine
Falcons [5] . Centre line of box denotes
median; bounds of box denote first and third quartiles. Crosses
indicate outlying points falling >1.5 times interquartile range
below the first quartile or above the third quartile; whiskers
extend to the most extreme data points not considered outliers. Red
dot denotes N -value for globally
fitted mixed guidance law. Silhouettes show typical values for
missiles [6] and predatory
flies [15] , [20] . b , c Trajectories
simulated under PN guidance at N ∈ {1, 2, 3}, in pursuit of ( b ) jinking ground target from hawk experiments, and
( c ) aerial target from falcon
experiments. Initial position of attacker as measured; initial track
angle directed at target to avoid bias. Coloured circles denote
collision. Grid spacing: 10 m. Fly icons redrawn from original
artwork in refs. [15] , [20] under CC BY 4.0 Full size image Whereas our Harris’ Hawks attacked jinking ground targets at N ≈ 1 (bootstrapped 95% CI for \(\tilde N\) : 0.81, 1.01), Peregrine Falcons have been found to operate at
significantly higher N -values against stationary
and manoeuvring targets mimicking typical prey behaviours (bootstrapped 95% CI for \(\tilde N\) : 1.76, 2.87). For falcons attacking stationary ground
targets [6] , the median \(\tilde N = 2.6\) is remarkably close to the well-known theoretical optimum of N = 3 for this case [7] . The same median was also
observed in falcons attacking manoeuvring aerial targets [6] , which is interesting because
a physics-based simulation study [3] has found that the catch success of model
falcons against erratically manoeuvring prey is maximized at N ≈ 3. Hence, the guidance system of Peregrine Falcons does appear
to be optimised in relation to their flight ecology. Is the same true of Harris’
Hawks? To answer this, we simulated the effect of parametrically varying N ∈ {1, 2, 3} in attacks on targets drawn from our experiments with hawks and falcons. Intriguingly, capture of the jinking target occurred soonest at N = 1 (Fig. 6b ), whereas capture of the gently manoeuvring target
used with falcons occurred soonest at N = 3
(Fig. 6c ). For these examples, at least,
the different N -values observed in hawks and
falcons therefore work best on the kinds of targets against which they were
observed. More generally, lower N -values cause
lower amplification of a jinking target’s twists and turns, reducing the extent to
which these throw the attacker off course (Fig. 6b ). This is especially important at close range, as the angular
effect of an evasive motion declines with distance. The guidance behaviour of
Harris’ Hawks is therefore appropriately tuned for close pursuit of the terrestrial
prey on which they specialise. We did not directly study the role of habitat clutter in this
experiment, but the clutter that is typical of the habitats in which hawks hunt
offers another possible functional account of why a mixed guidance law might be
advantageous. The intercept trajectories produced at high N -values work well in the open, but need not result in a feasible
path through clutter. In contrast, the tail-chase trajectories produced at low N -values, which the PP element of a mixed
guidance law reinforces, inherently cause a pursuer to follow the lead of its prey
through clutter. The same reasoning might also explain the behaviour of predatory
flies: the robber fly Holcocephala fusca intercepts prey in the open and operates at N ≈ 3
like a falcon, whereas the killer fly Coenosia
attenuata hunts in clutter and operates at a lower value of N ≈ 1.5, more like a hawk [15] . Hence, across two phyla
and five orders of magnitude of body mass, two aerial predators that intercept prey
in the open do so much like the guided missiles they resemble, whereas two that
closely pursue prey in clutter operate at lower feedback gain (Fig. 6a ). We therefore predict that, when comparing attack
trajectories phenomenologically, low N -values
will typify aerial, aquatic and cursorial predators that pursue agile prey through
clutter, whereas higher values of N ≈ 3 will
typify predators that intercept their prey in open environments. Experimental design We flew n = 5 captive-bred
Harris’ Hawks Parabuteo unicinctus (Supplementary Table 1 ), at an
unpredictably manoeuvring target simulating the jinking manoeuvres of a typical
prey item (Fig. 7 ). Tests with birds R
and F were conducted on a sloping open grassy field near Abergavenny, UK, from
October to December 2012; tests with birds A, J and S were conducted on another
sloping open grassy field in the same area, from July to September 2013. Each
pursuit was filmed using four S-PRI high-speed video cameras (Lake Image Systems
Ltd, Tring, UK) fitted with 28 mm f/2.8D lenses (Nikon Corporation, Tokyo,
Japan), recording RGB footage at 250 Hz (1280 × 1024 pixels; 0.002 s exposure). The cameras were manually post-triggered to give 8 s recording time, and were
calibrated as detailed below to enable three-dimensional (3D) reconstruction of
the trajectory of the hawk and the lure (see Videogrammetry). We continued
testing until we had obtained ≥20 flights for each bird, in which the lure was
intercepted successfully within view of the cameras. We recorded many other
flights in which the hawk failed to intercept the lure, but we do not analyse
them here because it is uncertain whether the hawk was locked on to its target
for the duration of those flights. To deal with the volume of data (~1 M frames
in total), and to ensure a balanced design, we determined to analyse only the
last 10 flights from each individual. All individuals therefore experienced a
training period of ≥10 successful flights before the set of flights that we
analysed. Fig. 7 Schematic of experimental design. Overhead view, with
shaded wedges denoting the overlapping fields of view of the
cameras. The bird began its attack from a perch positioned
behind the starting position of the lure (not to scale), which
followed a zigzagging course around a series of pulleys (red
circles). The lure began moving from one of three covered start
positions (grey ovals), and was then pulled around a randomised
subset of six from a total of ten pulleys. The lure was always
drawn around the two central pulleys (circled blue), but the
direction of its motion away from these pulleys was made
unpredictable by randomising which of the left or right outer
pulleys the lure was drawn towards (blue arrows). Outer pulleys
were covered by tunnels (black curves), to guide the lure and to
motivate chasing behaviour. The experimenter attempted to keep
the lure ahead of the hawk until the end of the course, by
controlling the speed of the lure. The lure’s start position was
randomised on each trial, as was the subset of outer pulleys
around which the lure was pulled, giving a total of 16 possible
courses for the lure to follow. Dummy lines were laid to avoid
the bird reading the course that had been laid ahead of the
flight. An illustrative lure trajectory is shown as a grey line. Blue dashed arrows denote sections where the lure’s direction of
travel was unpredictable; black dashed arrows denote sections of
the lure’s trajectory where the direction of travel might have
been anticipated if the bird had learned that the lure was
always pulled towards the central pulleys from the outer
pulleys Full size image Experimental protocol The hawks were fitted with a falconry harness (TrackPack, Marshall
Radio Telemetry, North Salt Lake, UT, USA), comprising a plastic mounting plate
held between the shoulders by a pair of Teflon ribbons drawn once around the
bird’s body in a figure-of-eight. The harness was fitted with two brightly
coloured 0.04-m-diameter polystyrene balls attached to the crossover point on
the breast and mounting plate on the back. The hawks were flown individually
from the top of the test area, taking off at will, as soon as the lure started
moving, from either a T-shaped perch, the falconer’s first, or a low tree
branch. A 0.1 m diameter food lure was attached by 100 m of kite line to an
electric winch (Expert Winch, Gliders Distribution, Newark, UK) that pulled the
lure at speed down a zigzagging course through a mown grassy field with a 1:10
slope (Fig. 7 ). The lure line was run
around a series of pulleys to generate abrupt changes in direction. We used ten
pulleys in total, six of which were built into tunnels to guide the lure and
motivate the hawks to chase the intermittently vanishing target. This allowed
the lure to be dragged along 16 alternative courses from three different
starting positions, switching direction four to six times on each course
(Fig. 7 ). We randomly selected which
course to use on each flight, laying dummy lines and placing covers over the
starting positions to prevent the birds anticipating the course. The lure was
always pulled towards the middle of the course at the outside pulleys, so it is
possible in principle that the hawks could have learned to anticipate the
direction of these switches. The lure could be pulled in either direction at the
middle pulleys, so the birds could not have learned to anticipate the direction
of these switches, unless by discriminating which line was under tension. The
birds were not motivated to continue chasing the lure if it was allowed to
outpace them, so the winch was controlled manually and stopped at the point of
capture to avoid harming the bird. Videogrammetry The cameras were calibrated on every test day by filming a
calibration object that was moved through the test volume in a range of
orientations. The calibration object comprised a 1.05-m long clear acrylic tube
with a coloured marker ball at each end. The pixel coordinates of the two marker
balls were tracked automatically (see below), and a self-calibrating bundle
adjustment was used to identify jointly optimal estimates of the camera
extrinsic and intrinsic parameters and the pose of the calibration object, by
solving the camera collinearity equations using a nonlinear least squares solver
in M atlab (The Mathworks Inc., Natick,
MA). Because lens distortions were minimal, we assumed a simple perspective
projection. Field measurements of camera position were used to specify initial
estimates of the extrinsic parameters to ensure convergence of the solver. Having first optimized the intrinsic parameters separately for each flight, we
ultimately fixed the principal distance of the cameras at 28.4 mm for all
flights, calculated as the mean for all cameras over all flights. This was done
on the basis that there was no systematic variation in the estimated principal
distance between cameras, so that the grand mean represents the best estimate of
the true value of this parameter. We established the error of our camera calibration by calculating
the standard deviation of the estimated distance between the end markers of the
calibration object over all of the frames. The camera calibration procedure
treats these markers as fixed points on a rigid body at 1.05 m spacing. Having
calibrated the cameras under this assumption, we then relaxed this rigid body
constraint by estimating the positions of the end markers independently, using
the same code that was subsequently used to estimate the position of the lure
and the markers on the bird. Because the calibration object was moved through
the test volume in a range of different positions and orientations, the standard
deviation of the estimated distance between its end markers provides an
isotropic estimate of the measurement error. Across trials, the standard
deviation of the estimated distance between the calibration object end markers
was 0.023 m, with 95% of the deviations from the mean falling on the interval
[−0.032, 0.036] m. It follows that the typical error of our camera calibration
is approximately three orders of magnitude smaller than the length of the
measurement volume. The pixel coordinates of the lure and the markers on the bird were
automatically identified using custom-written software in M atlab (The Mathworks Inc., Natick, MA). Tracking
of the lure and markers was done automatically using custom-written code in
M atlab . The user first created a
colour template by manually identifying the tracked object in a series of
specified video frames. A local search area was then defined around the marker,
and the software used the colour template to identify matching pixels within
this region of interest, updating the search area by centring it on the last
successfully tracked point. To identify matching pixels, the colour of each
pixel within the search area was compared with the distribution of the colour
template by computing its Mahalanobis distance. Any pixels with a Mahalanobis
distance below a set threshold were treated as candidate marker pixels, and the
centroid of the single largest contiguous group of candidate marker pixels was
assumed to correspond to the centroid of the marker itself. The software used a
Kalman filter to estimate the position of the marker if no marker was found, or
if the estimated position of the marker had moved too far between frames. Frames
in which the markers were not visible were treated as missing data. All
estimated marker positions were checked by the user and corrected manually if
necessary. We usually tracked only the bird’s breast marker, but used the back
marker for the whole flight if the breast marker was obscured. The trajectories
that we recorded were always close to planar, and we therefore projected them
onto the ground plane defined by the first and second principal components of
the lure’s path. All subsequent analysis was performed on this two-dimensional
(2D) projection of the data, which always captured >98% (typically >99.9%)
of the 3D variation in the bird’s measured position (Supplementary
Table 2 ). We defined the track
angle of the bird ( γ ) as the polar angle of
its velocity vector in the ground plane, and the line-of-sight angle ( λ ) as the polar angle of the vector from bird to
lure. We used cubic interpolation to fill in any missing data points, before
smoothing the 2D trajectories using quintic splines fitted at a tolerance
designed to remove a root mean square error matching the diameter of the marker
or lure. Finally, we differentiated and evaluated the splines analytically to
estimate the velocity and acceleration of the bird and lure at 16 kHz, which
ensured an adequately small integration step size for our simulations. Simulations of guidance behaviour We simulated the hawks’ measured flight trajectories by predicting
the hawk’s turning rate \(\dot \gamma \left( t \right)\) using (i) a proportional pursuit (PP) guidance law \(\dot \gamma (t) = - K\delta (t - \tau )\) , where δ = γ − λ is the
deviation angle and K is a guidance constant;
(ii) a proportional navigation (PN) guidance law \(\dot \gamma (t) = N\dot \lambda (t - \tau )\) , where \(\dot \lambda (t)\) is the line-of-sight rate and N is a guidance constant called the navigation constant; (iii) a
mixed guidance law combining PP and PN elements to command turning as \(\dot \gamma (t) = N\dot \lambda (t - \tau ) - K\delta (t - \tau )\) . We used the same simulation algorithm as in our previous work
on falcons [6] , given knowledge only of the hawk’s initial
track angle and initial position, and given the complete time history of the
lure’s motion, always matching the hawk’s simulated groundspeed to its measured
groundspeed (see Supplementary Data 1 for raw trajectory data and simulation code). Writing the simulated position vector of the pursuer as x P , and the measured position
vector of the target as \({\hat{\mathbf{x}}}_{\mathrm{T}}\) , we define the line-of-sight vector ( r ) as: 
    r = x̂_T - x_P
 (1) and the closing velocity ( v C ) as: 
    v_C = v_P - v̂_T
 (2) The deviation angle ( δ ) is given
in vector form as: 
    δ = ( cos^ - 1r·v_P/| r| | v_P|)( r×v_P/| r×v_P|)
 (3) whilst the line-of-sight rate ( ω )
is given in vector form as: 
    ω = r×(  - v_C)/| r|^2
 (4) Under PP, the pursuer’s turning at time t is commanded at a rate proportional to the deviation angle at
time t − τ , such that its commanded centripetal acceleration is given
by: 
    a_P(t) = - Kδ(t - τ ) ×v_P(t)
 (5) where K is a guidance constant. Under PN, the pursuer’s turning is commanded at a rate proportional to the
line-of-sight rate, such that its commanded centripetal acceleration is given
by: 
    a_P(t) = Nω(t - τ ) ×v_P(t)
 (6) where N is a guidance constant
called the navigation constant. Under the mixed guidance law, these PP and PN
elements are combined to command the pursuer’s centripetal acceleration
as: 
    a_P(t) = Nω(t - τ ) ×v_P(t) - Kδ(t - τ ) ×v_P(t)
 (7) In our simulations, the preceding equations are implemented in
discrete time, and coupled by the difference equations: 
    x_P_n + 1 = x_Pn + Δt v_Pn
 (8) 
    v_P_n + 1 = v̂_P_n + 1v_Pn + Δt a_Pn/| v_Pn + Δt a_Pn|
 (9) where \(\hat v_{\mathrm{P}} = \left| {{\hat{\bf{v}}}_{\mathrm{P}}} \right|\) denotes the actual measured speed of the pursuer, and where
the subscript notation indicates the values of the variables at successive time
steps, such that t n +1 = t n + Δ t . The step
size Δ t in our simulations was made small
enough to guarantee the accuracy of the fitted guidance parameters and
prediction error (see below) to the level of precision at which they are
reported (Δ t = 6.25 × 10 −5 s). The first of
these difference equations advances the simulated position of the pursuer from x P n to x P n +1 using the simulated velocity v P n . The second difference equation advances the
simulated velocity of the attacker from v P n to v P n +1 by using the commanded centripetal acceleration a P n to rotate v P n , but then scales the rotated vector to match the
measured speed of the attacker ( \(\hat v_{{\mathrm{P}}_{n + 1}}\) ). Code implementing these equations of motion is provided in
Supplementary Data 1 . System identification We fitted the guidance constant K or N and time delay τ under the PP and PN guidance laws for
each flight independently, modelling every possible delay τ ≤ τ max at a spacing corresponding to the
0.004 s inter-frame interval where τ max = 0.4 s. Taking time t = 0 as take-off, we simulated the bird’s flight
trajectory from t = τ max to the point of intercept or first
near-miss. This ensured that the same section of flight was analysed for all
time delays. For each value of τ , we used a
Nelder-Mead simplex algorithm in M atlab to
find the value of K or N that minimised the prediction error ε , defined as the mean absolute distance between
the measured ( \({\hat{\bf{x}}}_{\mathrm{P}}\) ) and simulated ( x P ) positions of the bird at each time
point: 
    ε = 1/k∑_n = 1^k  | x_Pn - x̂_Pn|
 (10) We then optimized τ by selecting
the value that minimised the prediction error ε over all of the fitted values of τ . We fitted the mixed guidance law globally to all of the flights,
identifying the unique combination of the guidance constants K or N and the
time delay τ that minimised the median
prediction error \(\tilde \varepsilon\) over all flights. This was done through an exhaustive search
of the prediction error ε for values of K and N on the interval [0, 2] at 0.1 spacing, and values of τ on the interval [0, 0.1] at 0.004 s spacing,
these values being chosen in light of the independently fitted optima for PP and
PN. 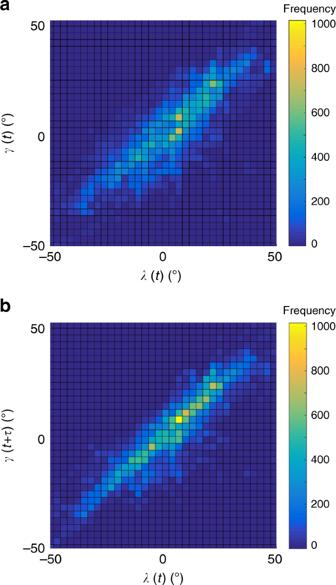Fig. 3 Correlation of track angle and line-of-sight angle. Each
figure panel plots a two-dimensional histogram of track angleγagainst line-of-sight
angleλfor all sample points
over all flights:ano delay
betweenγ(t) andλ(t);btrack angleγlagged byτ= 0.16 s delay, representing the median value
of the delay at which the correlation betweenγ(t+τ) andλ(t) was maximised for each flight. The linear
association inbindicates that
the attack trajectories of the hawks approximated a delayed pure
pursuit course Finally, to improve the precision of the estimates, we refined the search by
a factor of 10 in the vicinity of the identified optimum. Statistical analysis To test whether the hawks’ trajectories followed a pure pursuit
course, we compared the track angle γ ( t ) at time t with the angle of the line-of-sight to target λ ( t − τ ) at delay τ , by binning all of the data in a two-dimensional
(2D) histogram. 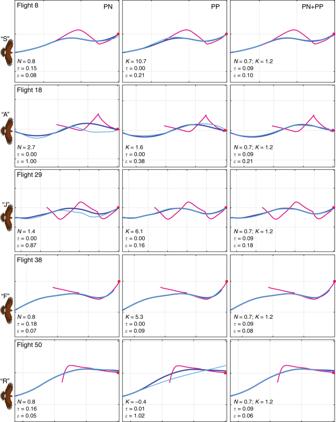Fig. 4 Comparison of measured and simulated attack
trajectories. Panels display measured attack trajectories (dark
blue) and best-fitting simulations (light blue) for each Harris’
Hawk in pursuit of the lure (magenta), arranged by individual
bird (rows) and by guidance law (columns; PN: proportional
navigation; PP: proportional pursuit; PN + PP: mixed guidance
law). The time delayτ(s)
and guidance constantK(s−1) orNare independently fitted to each
flight for PP and PN, but are globally fitted to all flights for
the mixed guidance law. For each bird, we display the flight
with the least prediction errorε(m) under the mixed guidance law (excluding
flights <20 m), to best show the complementarity of its PN
and PP elements: whilst all flights are well-modelled by the
globally fitted mixed guidance law, some are not well-modelled
by PN or PP, despite these being independently fitted to each
flight; see Supplementary Figs.1–9for all other flights. Grid spacing: 10 m We also computed the cross-correlation sequence of γ and λ independently for each flight. We analysed the statistical distributions of the
fitted guidance parameters and prediction error across all 50 flights, reporting
their median (denoted by a tilde) and interquartile range (IQR) for robustness
against outliers and skew. Where relevant, we also report bootstrapped 95%
confidence intervals (CIs) for the medians. These were computed using the
bias-corrected and accelerated percentile method over
10 6 iterations, using a customised version of the
corresponding function in M atlab to
implement multistage resampling by individual as appropriate to the structure of
the data. The hierarchical structure of the published data on Peregrine
Falcons [4] was too complicated to handle by this method,
so each attack pass had to be treated as independent when bootstrapping these
data. 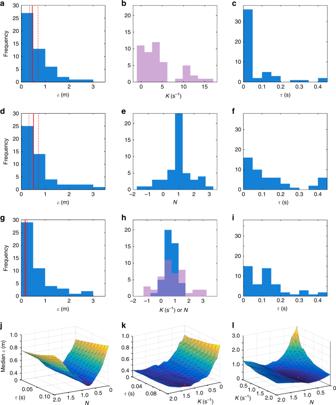Fig. 5 Model parameters and fit under each guidance law.a–cproportional pursuit (PP), fitted
independently to each flight;d–fproportional navigation (PN), fitted independently to each
flight;g–imixed (PP + PN) guidance law, fitted
independently to each flight;j–lmixed
(PP + PN) guidance law, fitted globally to all flights.a,d,ghistograms
showing the prediction errorεof the best-fitting model for each flight,
where the solid and dashed red lines denote the median
prediction error\(\tilde \varepsilon\)and its bootstrapped 95% confidence interval;b,e,hhistograms
showing the best-fitting guidance constantK(magenta) and/orN(blue) for each flight;c,f,ihistograms
showing the best-fitting delayτfor each flight.j–lSurface
plots showing how median prediction error\(\tilde \varepsilon\)for all flights varies as a function of each
pair of the parametersN,Kandτof the mixed guidance law,
holding the third parameter constant at its best-fitting value.
Surface colour denotes surface height; red dot denotes location
of global optimum A two-tailed Kruskal–Wallis test was used to test for differences in the
mean ranks of the fitted guidance constants between individuals, with post hoc
testing done using Tukey’s HSD test at α = 0.05. 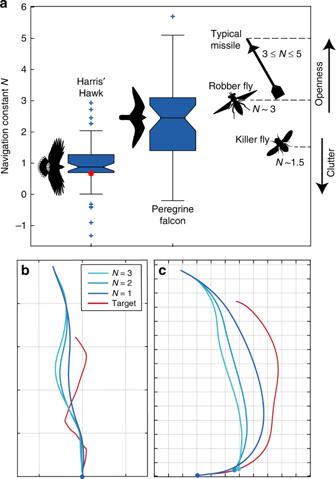Fig. 6 Comparative analysis of guidance behaviour.aBox-and-whisker plots comparingN-values for PN guidance
models fitted independently to 50 flights from Harris’ Hawks (this
paper) and 42 flights from Peregrine
Falcons5. Centre line of box denotes
median; bounds of box denote first and third quartiles. Crosses
indicate outlying points falling >1.5 times interquartile range
below the first quartile or above the third quartile; whiskers
extend to the most extreme data points not considered outliers. Red
dot denotesN-value for globally
fitted mixed guidance law. Silhouettes show typical values for
missiles6and predatory
flies15,20.b,cTrajectories
simulated under PN guidance atN∈{1, 2, 3}, in pursuit of (b) jinking ground target from hawk experiments, and
(c) aerial target from falcon
experiments. Initial position of attacker as measured; initial track
angle directed at target to avoid bias. Coloured circles denote
collision. Grid spacing: 10 m. Fly icons redrawn from original
artwork in refs.15,20under CC BY 4.0 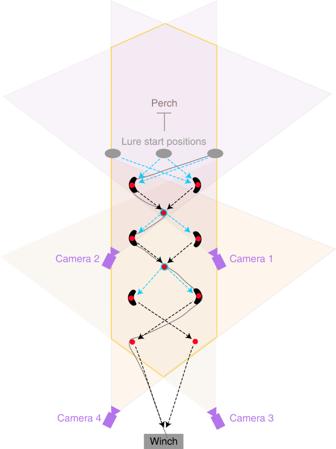Fig. 7 Schematic of experimental design. Overhead view, with
shaded wedges denoting the overlapping fields of view of the
cameras. The bird began its attack from a perch positioned
behind the starting position of the lure (not to scale), which
followed a zigzagging course around a series of pulleys (red
circles). The lure began moving from one of three covered start
positions (grey ovals), and was then pulled around a randomised
subset of six from a total of ten pulleys. The lure was always
drawn around the two central pulleys (circled blue), but the
direction of its motion away from these pulleys was made
unpredictable by randomising which of the left or right outer
pulleys the lure was drawn towards (blue arrows). Outer pulleys
were covered by tunnels (black curves), to guide the lure and to
motivate chasing behaviour. The experimenter attempted to keep
the lure ahead of the hawk until the end of the course, by
controlling the speed of the lure. The lure’s start position was
randomised on each trial, as was the subset of outer pulleys
around which the lure was pulled, giving a total of 16 possible
courses for the lure to follow. Dummy lines were laid to avoid
the bird reading the course that had been laid ahead of the
flight. An illustrative lure trajectory is shown as a grey line.
Blue dashed arrows denote sections where the lure’s direction of
travel was unpredictable; black dashed arrows denote sections of
the lure’s trajectory where the direction of travel might have
been anticipated if the bird had learned that the lure was
always pulled towards the central pulleys from the outer
pulleys Ethics statement We affirm that we have complied with all relevant ethical
regulations for animal testing and research. The study protocol was approved by
the United States Air Force, Surgeon General’s Human and Animal Research Panel,
and by the Local Ethical Review Committee of the University of Oxford’s
Department of Zoology, and was considered not to pose any significant risk of
causing pain, suffering, damage or lasting harm to the animals. Reporting summary Further information on research design is available in
the Nature Research Reporting
Summary linked to this article.